Whole-genome sequence-based analysis of thyroid function Normal thyroid function is essential for health, but its genetic architecture remains poorly understood. Here, for the heritable thyroid traits thyrotropin (TSH) and free thyroxine (FT4), we analyse whole-genome sequence data from the UK10K project ( N =2,287). Using additional whole-genome sequence and deeply imputed data sets, we report meta-analysis results for common variants (MAF≥1%) associated with TSH and FT4 ( N =16,335). For TSH, we identify a novel variant in SYN2 (MAF=23.5%, P =6.15 × 10 −9 ) and a new independent variant in PDE8B (MAF=10.4%, P =5.94 × 10 −14 ). For FT4, we report a low-frequency variant near B4GALT6/SLC25A52 (MAF=3.2%, P =1.27 × 10 −9 ) tagging a rare TTR variant (MAF=0.4%, P =2.14 × 10 −11 ). All common variants explain ≥20% of the variance in TSH and FT4. Analysis of rare variants (MAF<1%) using sequence kernel association testing reveals a novel association with FT4 in NRG1. Our results demonstrate that increased coverage in whole-genome sequence association studies identifies novel variants associated with thyroid function. Thyroid hormones have fundamental but diverse physiological roles in vertebrate physiology, ranging from induction of metamorphosis in amphibians to photoperiodic regulation of seasonal breeding in birds [1] . In humans, they are essential for adult health and childhood development [2] , [3] and levothyroxine is one of the commonest drugs prescribed worldwide. Clinically, thyroid function is assessed by measuring circulating concentrations of free thyroxine (FT4) and the pituitary hormone thyrotropin (TSH); the complex inverse relationship between them renders TSH the more sensitive marker of thyroid status [4] . Even small differences in TSH and FT4, within the normal population reference range, are associated with a wide range of clinical parameters, including blood pressure, lipids and cardiovascular mortality, as well as obesity, bone mineral density and lifetime cancer risk [5] . Twin and family studies estimate the heritability of TSH and FT4 as up to 65% [6] . Genome-wide association studies (GWAS) identified common variants associated with TSH and FT4 [7] , [8] , [9] ; in a recent HapMap-based meta-analysis [10] , we identified 19 loci associated with TSH and 4 with FT4. However, these accounted for only 5.6% of the variance in TSH and 2.3% in FT4. Therefore, most of the heritability of these important traits remains unexplained. The unidentified genetic component of variance might be explained by common variants poorly tagged by markers assessed in previous studies, or those with small effects. However, rarer variants within the minor allele frequency (MAF) spectrum might also account for a substantial proportion of the missing heritability as has been proposed for many polygenic traits [11] . These variants, although individually rare (MAF<1%), are collectively frequent, and while their effects may be insufficient to produce clear familial aggregation, effect sizes for individual variants are potentially much greater than those observed for common variants. In addition, a greater understanding of the relative proportion of thyroid function explained by common variants is now possible with the availability of whole-genome sequencing (WGS) and this is essential to refine future research and analysis strategies when appraising the genetic architecture of thyroid function. In this study, the first to utilize WGS to examine the genetic architecture of TSH and FT4, we perform single-point association analysis in two discovery cohorts in the UK10K project with WGS data available and a meta-analysis using genome wide association data (GWAS) with deep imputation from five additional data sets. We report three new loci associated with thyroid function in healthy individuals, undertake quantitative trait loci and DNA methylation analyses to further study these relationships and undertake genome-wide complex trait analyses (GCTA) [12] to assess the contributions of common variants (MAF≥1%) to variance in thyroid function. We also explore whether there is a shared polygenic basis between TSH and FT4. In individuals with WGS data, we perform sequence kernel-based association testing (SKAT) analysis to identify regions of the genome where rare variants have the strongest association with thyroid function and identify a novel locus associated with FT4. The results demonstrate that WGS-based analyses can identify rare functional variants and associations derived from rare aggregates. Larger meta-analyses of studies with WGS data are now required to identify additional common and rare variants, which may explain the missing heritability of thyroid function. Single-point association analysis In the discovery study, using a meta-analysis of WGS data from the Avon Longitudinal Study of Parents and Children (ALSPAC) and TwinsUK cohorts ( N =2,287) analysing up to 8,816,734 markers ( Supplementary Tables 1 and 2 ; Supplementary Methods ), we find associations at two previously described loci for TSH. These are NR3C2 (rs11728154; MAF=21.0%, B =0.21, s.e.=0.037, P =8.21 × 10 −9 ; r 2 =0.99 with the previously reported rs10028213) and FOXE1 (rs1877431; MAF=39.5%, B =−0.19, s.e.=0.030, P =2.29 × 10 −10 ; r 2 =0.99 with the previously reported rs965513). We find one borderline signal (between P =5.0 × 10 −08 and P =1.17 × 10 −08 ) at a novel locus FAM222A (rs11067829; MAF=18.3%, B =0.210, s.e.=0.038, P =3.73 × 10 −8 ; Supplementary Figs 1a and 2 ; Supplementary Table 3 ). No variants show genome-wide significant association for FT4 ( Supplementary Figs 1a and 3 ). 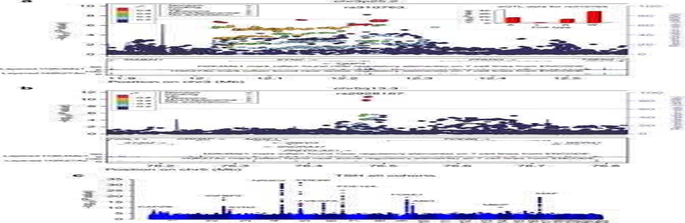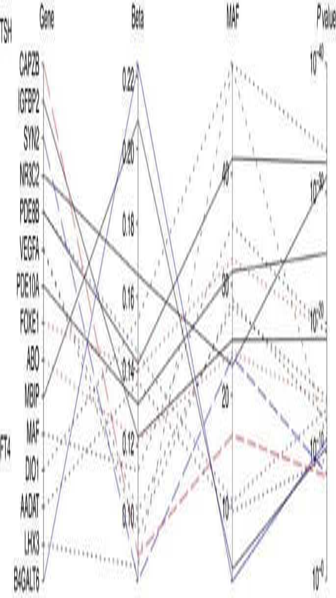Figure 3: Overview of our findings of SNPs associated with TSH and FT4. Blue coloured lines represent a novel signal identified in this meta-analysis. Red lines represent heterogeneity observed between the different cohorts in the association between the variant and TSH. - - - Indicates responsiveness observed to levothyroxine. — — Indicates observed eQTL or meQTL associations. Figure 1: Regional and genome-wide association plots for TSH. (a) Regional association plot showing genome-wide significant locus for serum TSH at theSYN2, TIMP4gene region. Inset isin vitroexpression QTL data for the lead SNP rs310763 in adipose cells (A), lymphoblastoid cell lines (L), skin cells (S) and whole blood (W). Dotted line denotes genome-wide significance threshold. (b) Regional association plot after conditional analysis on rs2046045 inPDE8Bshowing our novel association with TSH at rs2928167 inPDE8Bremained genome-wide significant. (c) Annotated Manhattan plot from the overall analysis for serum TSH levels. SNPs (MAF>1%) are plotted on thexaxis according to their position on each chromosome against association with TSH on theyaxis (shown as −log10(Pvalue)). The loci are regarded as genome-wide significant atP<5 × 10−8. Variants with 1%<MAF<5% are shown as open diamond symbols. Common SNPs (MAF>5%) are shown as solid circles with those present in Hapmap II reference panels in grey and those derived from WGS or deeply imputed using WGS and 1000 genomes reference panels in blue. SNPs shown as a red asterisk represent novel genome-wide significant findings. In a meta-analysis of the discovery cohorts and five additional cohorts, we find associations for 13 SNPs at 11 loci for TSH ( N =16,335) of which 11 loci have been identified previously and 4 SNPs at 4 loci for FT4 ( N =13,651) of which 3 have been identified previously ( Table 1 ; Figs 1a–c , 2a,b and 3 ; Supplementary Figs 1b and 3–6 ). Table 1 Independent SNPs with MAF≥1% associated with serum TSH and FT4 levels in the overall meta-analysis. Full size table Figure 1: Regional and genome-wide association plots for TSH. ( a ) Regional association plot showing genome-wide significant locus for serum TSH at the SYN2, TIMP4 gene region. Inset is in vitro expression QTL data for the lead SNP rs310763 in adipose cells (A), lymphoblastoid cell lines (L), skin cells (S) and whole blood (W). Dotted line denotes genome-wide significance threshold. ( b ) Regional association plot after conditional analysis on rs2046045 in PDE8B showing our novel association with TSH at rs2928167 in PDE8B remained genome-wide significant. ( c ) Annotated Manhattan plot from the overall analysis for serum TSH levels. SNPs (MAF>1%) are plotted on the x axis according to their position on each chromosome against association with TSH on the y axis (shown as −log 10 ( P value)). The loci are regarded as genome-wide significant at P <5 × 10 −8 . Variants with 1%<MAF<5% are shown as open diamond symbols. Common SNPs (MAF>5%) are shown as solid circles with those present in Hapmap II reference panels in grey and those derived from WGS or deeply imputed using WGS and 1000 genomes reference panels in blue. 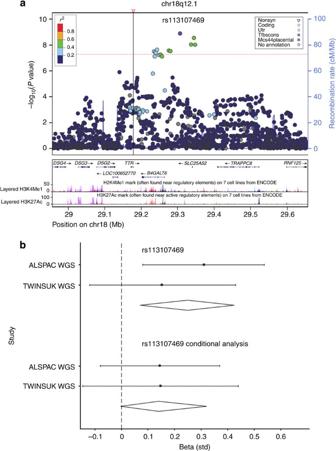SNPs shown as a red asterisk represent novel genome-wide significant findings. Figure 2: Regional and conditional plots for FT4. (a) Regional association plot showing genome-wide significant locus for serum FT4 at theB4GALT6, SLC25A52region (overall meta-analysis).∇shows the location of the Thr139Met substitution (rs28933981; MAF=0.4%) inTTR. Dotted red line denotes genome-wide significance threshold. (b) Forest plots of WGS association data for rs113107469 in the WGS discovery studies and meta-analysis, and below is the illustrating loss of signal on conditioning with rs28933981. Squares represent beta estimate and error bars represent 95% CI. Full size image Figure 2: Regional and conditional plots for FT4. ( a ) Regional association plot showing genome-wide significant locus for serum FT4 at the B4GALT6, SLC25A52 region (overall meta-analysis). ∇ shows the location of the Thr139Met substitution (rs28933981; MAF=0.4%) in TTR . Dotted red line denotes genome-wide significance threshold. ( b ) Forest plots of WGS association data for rs113107469 in the WGS discovery studies and meta-analysis, and below is the illustrating loss of signal on conditioning with rs28933981. Squares represent beta estimate and error bars represent 95% CI. Full size image Figure 3: Overview of our findings of SNPs associated with TSH and FT4. Blue coloured lines represent a novel signal identified in this meta-analysis. Red lines represent heterogeneity observed between the different cohorts in the association between the variant and TSH. - - - Indicates responsiveness observed to levothyroxine. — — Indicates observed eQTL or meQTL associations. 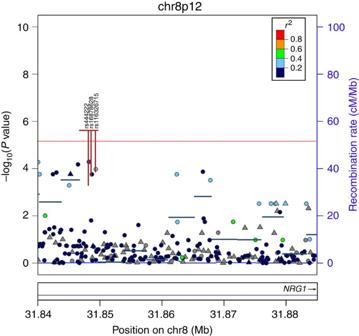Figure 4: Plots showingNRG1region with significant associations with FT4 from SKAT analysis. Horizontal bar represents SKAT variant bins. (·)=single-point association data. Vertical lines in the bin (|) highlight rare variants that contribute to the association with a contribution proportional to the length of the line (that is, removal of the variant from the analysis causes the significance to fall to the level shown). Full size image To determine whether our identified associations at established loci represented previous association signals, we analysed the linkage disequilibrium (LD) between the strongest associated variants from this study and those from our previous study [10] ( Supplementary Table 4 ). The top variants from loci in both studies were in strong LD ( r 2 >0.6), apart from MBIP and FOXE1 , although these were in strong LD with variants previously associated with TSH by others [8] . Two SNPs associated with TSH in our study are novel, one at SYN2 (rs310763; MAF=23.5%, B =0.082, s.e.=0.014, P =6.15 × 10 −9 ; Fig. 1a–c ). SYN2 is a member of a family of neuron-specific phosphoproteins involved in the regulation of neurotransmitter release with expression in the pituitary and hypothalamus ( http://biogps.org/#goto=genereport&id=6854 ). We also identify one novel variant at PDE8B (MAF=10.4%, B =−0.145, s.e.=0.019, P =5.94 × 10 −14 ) in linkage equilibrium ( r 2 =0.002, D ′=0.17) with the previously described variant rs6885099 (ref. 10 ) and independent from our top SNP rs2046045 ( P =1.93 × 10 −11 ) after conditional analysis. In the overall meta-analysis, we are unable to replicate the association between FAM222A and TSH in the discovery analysis ( B =0.014, s.e.=0.015, P =0.378); however, we observe evidence of heterogeneity between cohorts (test for heterogeneity P =4.70 × 10 −6 ; Supplementary Table 5 ), so potentially this locus may find support in future WGS studies. In our meta-analysis, we also identify four SNPs associated with FT4, three at previously established loci ( DIO1 , LHX3 and AADAT ; Table 1 ; Fig. 3 ; Supplementary Figs 1b, 4e and 6 ; Supplementary Table 4 ). We find a novel uncommon variant at B4GALT6 / SLC25A52 associated with FT4 (rs113107469; MAF=3.20%, B =0.225, s.e.=0.037, P= 1.27 × 10 −9 ; Fig. 2a ). B4GALT6 is in the ceramide metabolic pathway, which inhibits cyclic AMP production in TSH-stimulated cells. However, the B4GALT6 signal (rs113107469) is in weak LD ( r 2 <0.1, D ′=0.66) with the Thr139Met substitution (rs28933981; MAF=0.4%) and it may therefore be a marker for this functional change in TTR . The Thr139Met substitution was associated with FT4 levels in our single-point meta-analysis ( P =2.14 × 10 −11 ), however, was not originally observed as the MAF was lower than our 1% threshold. Conditional analysis of the TTR region using rs28933981 as the conditioning marker in the ALSPAC WGS cohort reveals no evidence of association between rs113107469 in B4GALT6 and FT4 ( P =0.124; Fig. 2b ). Analysis using direct genotyping in the ALSPAC WGS and replication cohorts confirms the effect of the Thr139Met substitution on FT4 levels. Here, 0.79% of children were heterozygous for the Thr139Met substitution, which is positively associated with FT4 ( B =1.70, s.e.=0.17, 95% CI 1.37, 2.03, P =3.89 × 10 −24 ). In the ALSPAC replication data set, rs113107469 in B4GALT6 was also positively associated with FT4 ( P =0.0002); however, when conditioned on the Thr139Met substitution there was no longer any evidence of association ( P =0.20). The Thr139Met substitution also appears to be functional: this mutation has increased protein stability compared with wild-type transthyretin (TTR) [13] , [14] and tighter binding of thyroxine [14] , resulting in a twofold increase in thyroxine-binding affinity [15] , [16] . Further details of the likely genes related to all our observed independent novel signals are shown in Supplementary Table 6 . Expression quantitative trait locus analysis Expression quantitative trait locus (eQTL) analysis [17] , [18] reveals that our SYN2 variant modulates SYN2 transcription in adipose, skin and whole-blood cells, but not lymphoblastoid cell lines ( Supplementary Table 7 ). Furthermore, bioinformatics analysis suggests that the C-allele at rs310763 attenuates an EGR1 regulatory motif [19] . EGR1 is expressed in thyrocytes, regulates pituitary development [20] , [21] and may influence thyroid status via LHX3 promotor activity [20] . Several other variants in the SYN2 gene region are in strong LD ( r 2 >0.8) with rs310763, including the non-synonymous coding variant rs794999. Although predicted to be benign (PolyPhen-2 score=0.002 (ref. 22 )), rs794999 is located in a DNase hypersensitivity cluster [23] , influences four predicted regulatory motifs [19] and appears to be under evolutionary constraint [24] , [25] . SNPs identified in our study, or those in LD, also showed strong eQTL associations with PDE8B ( P =8.69 × 10 −27 ), FOXE1 ( P= 9.10 × 10 −54 ) and AADAT ( P =7.86 × 10 −9 ) gene expressions ( Supplementary Table 7 ). DNA methylation analysis To further explore cis -regulatory effects of variants identified in our study, we carried out analysis of DNA methylation profiles in whole-blood samples in 279 individuals from the TwinsUK cohort. We find evidence for a methylation quantitative trait locus (meQTL) at the novel TSH-associated variant rs2928167 in PDE8B ( P =4.38 × 10 −7 ; Supplementary Table 8 ), which are also eQTLs in multiple tissues ( Supplementary Table 7 ). Recently, meQTL effects using the same probe (cg16418800) in adipose tissue also identified a peak signal at rs2359775 ( P =6 × 10 −15 ), which is in LD with rs2928167 ( r 2 =0.5). We find that variants in ABO ( P =2.02 × 10 −23 ) and AADAT ( P =1.80 × 10 −8 ) also show strong evidence for cis -meQTL effects ( Supplementary Table 8 ). In additional analyses in 745 ALSPAC children, we find strong meQTL associations for rs2359775 in PDE8B ( P =3.03 × 10 −28 ) and variants in ABO ( P =1.01 × 10 −101 ) and AADAT ( P =4.18 × 10 −34 ) ( Supplementary Table 8 ). SKAT analysis Tests of the association between aggregates of rare variants (MAF<1%) in the WGS cohorts were restricted to genes relevant to thyroid function. We find no evidence of association from SKAT analyses with TSH, however, for FT4 we identify one SKAT bin with multiple-testing-corrected evidence for association ( P ≤1.55 × 10 −5 ) in NRG1 ( P =2.53 × 10 −6 ; Fig. 4 ; Supplementary Table 9 ). NRG1 is a glycoprotein that interacts with the NEU/ERBB2 receptor tyrosine kinase, and is critical in organ development. Figure 4: Plots showing NRG1 region with significant associations with FT4 from SKAT analysis. Horizontal bar represents SKAT variant bins. (·)=single-point association data. Vertical lines in the bin (|) highlight rare variants that contribute to the association with a contribution proportional to the length of the line (that is, removal of the variant from the analysis causes the significance to fall to the level shown). Full size image GCTA and polygenic score analysis SNPs were thinned to a set of 2,203,581 approximately independent SNPs with an LD threshold of r 2 >0.2, a window size of 5,000 SNPs and step of 1,000 SNPs. A genomic relationship matrix was then generated for unrelated individuals. We fitted linear mixed-effect models and estimate that all assessed common SNPs (MAF>1%) explain 24% (95% CI 19, 29) and 20% (95% CI 14, 26) of TSH and FT4 variance, respectively ( P ≤0.0001; Supplementary Table 10 ). Polygenic score analyses [21] based on SNPs with P values under a fixed threshold do not detect evidence of a polygenic signal for TSH or FT4, nor of a shared polygenic basis between thyroid function and key metabolic outcomes. However, a genetic score based on 67 SNPs previously associated with thyroid function in GWAS [8] , [10] , [26] shows strong evidence of association with TSH ( P =7.9 × 10 −20 ) and FT4 ( P =2.7 × 10 −4 ) and we observe evidence of shared genetic pathways with TSH associated with the FT4 gene score ( P =7.0 × 10 −4 ). These 67 SNPs explain 7.1% (95% CI 5.2, 9.0) of the variance in TSH and 1.9% (95% CI 1.1, 3.0) of the variance in FT4. Taken together, this suggests that many loci underlying thyroid function remain unknown. Chemogenomic analysis We undertook a database analysis of differential gene expression in cultured cells in response to hormone stimulation. We find SYN2 (rank 64 of 22283 (HL60 cells)) rates highest among the genes studied in the experiment, providing strong support for the role of this newly discovered locus in thyroid metabolism. Two other genes, NRG1 and CAPZB , also show evidence of levothyroxine responsiveness in at least one cell line [27] on the basis of a genome-wide differential expression and rank in the top 5th percentile ( Supplementary Table 11 ). Publicly available data on altered SYN2 expression in brain, limb and tail from control and levothyroxine-treated Xenopus laevis during metamorphosis also provide evidence for the relevance of SYN2 in thyroid function [28] . In this study, we demonstrate the utility of WGS data (and SNP array data when deeply imputed to WGS reference panels) in appraising the genetic architecture of thyroid function. Using WGS data, we identify a rare functional variant in TTR that appears to drive the observed association between an uncommon novel variant near B4GALT6 and FT4, and we demonstrate a novel association with FT4 arising from rare aggregates in NRG1 . We also show that common variants collectively account for over 20% of the variance in TSH and FT4, a substantial advance on using only the ‘top SNPs’ from earlier GWA studies [10] . Taken together, this work indicates that both common variants with modest effects and rare variants with larger effects might explain a substantial proportion of the missing heritability of thyroid function, but larger studies are required to identify these variants. Studies including individuals with subclinical thyroid disease, particularly those who are negative for thyroid autoantibodies, may be particularly rewarding, as rare genetic variants with large effect sizes may be associated with serum TSH and FT4 concentrations outside the inclusion ranges we used and therefore would not be detected in our analyses. Such endeavours are clinically relevant, as there has been a dramatic increase in levothyroxine prescribing for borderline TSH levels [29] . At least three loci identified in this study show evidence of responsiveness to levothyroxine in cell line models, underscoring that borderline TSH levels often reflect the influence of genetic variation rather than overt autoimmune thyroid disease, in which case thyroid hormone replacement may not be appropriate. Our results indicate that further investigation of TSH heterogeneity at the population level is necessary. Cohorts Seven populations were used in this study. They are known as the TwinsUK WGS cohort, the TwinsUK GWAS cohort, the ALSPAC WGS cohort, the ALSPAC GWAS cohort, the SardiNIA cohort, the ValBorbera cohort and the Busselton Health Study cohort. Summary statistics of each cohort and full descriptions are given in Supplementary Methods , Supplementary Tables 1 and 2 . All human research was approved by the relevant institutional ethics committees. WGS data generation Low-read depth WGS was performed in the TwinsUK and ALSPAC as part of the UK10K project. The SardiNIA cohort also had WGS data available (see Supplementary Methods ). Statistical analysis An inverse normal transformation was applied to each trait within each cohort. Age, age 2 , gender and any other cohort-specific variables ( Supplementary Table 1 ) were applied as covariates. Genotype imputation was performed for relevant cohorts using the IMPUTE [30] , MaCH [31] or Minimac [32] software packages, with poorly imputed variants excluded. See Supplementary Table 1 for cohort-specific details. Single-point association analysis Association analysis within each cohort was performed using the SNPTEST v2 (ref. 33 ), GEMMA (genome-wide efficient mixed model association) [34] , EPACTS (efficient and parallelizable association container toolbox) or ProbABEL [35] software packages. Cohort-specific quality control filters relating to call rate and Hardy–Weinberg equilibrium were applied ( Supplementary Table 1 ). In our analysis, we assessed the change in standardized thyroid measure by allele using a MAF threshold ≥1% and a genome-wide significance threshold of P =1.17 × 10 −08 (ref. 36 ). Meta-analyses were performed using the GWAMA (genome-wide association meta analysis) software [37] , which was used to perform fixed-effect meta-analyses using estimates of the allelic effect size and s.e. Two meta-analyses were performed for each phenotype: a meta-analysis of the two UK10K WGS cohorts and a meta-analysis of all seven cohorts. The ValBorbera cohort does not have FT4 phenotype data, so this cohort was not included in the meta-analyses for this phenotype. In the meta-analyses, any variants that were missing from >2 cohorts or with a combined MAF ≤1% were excluded. However, in the discovery analyses, a MAF of 0.5% in either cohort was accepted to prevent marginal MAF dropouts; the MAF <1% exclusion was then applied during the meta-analysis. Conditional analysis A conditional analysis was performed to identify independent association signals. Each study re-analysed significant loci using the lead SNP identified in the primary analysis ( Table 1 ) as the conditioning marker. In cohorts where the lead SNP was not available, the best proxy was included ( r 2 >0.8). A meta-analysis was then performed on these conditional results, using the same methods and filters as described above. The standard genome-wide significant cut-off ( P <5 × 10 −8 ) was used to identify secondary associations. Estimation of phenotypic variance explained by genetic variants We undertook GCTA using WGS data in the ALSPAC and TwinsUK discovery cohorts and data from the SardiNIA and Busselton cohorts to estimate the variance explained by all common SNPs (MAF>1%) in the genome for TSH and FT4, using the GCTA method of Yang et al . [12] We fitted linear mixed-effect models to estimate the phenotypic variance attributable to the common SNPs ( h g 2 ). In these data sets, SNPs were thinned to a set of 2,203,581 approximately independent SNPs using the –indep-pairwise option in PLINK with an LD threshold of r 2 >0.2, window size of 5,000 SNPs and step of 1,000 SNPs. A genomic relationship matrix was generated for unrelated individuals, namely, those with genomic correlation <0.025. Estimates were calculated on SNPs filtered for Hardy–Weinberg equilibrium P value ≥1 × 10 −6 and MAF ≥0.01. The genetic and residual variance components were estimated by the restricted maximum likelihood (REML) procedure for different MAF thresholds and for SNPs within a 250 kb window of known markers of thyroid function. Expression quantitative trait loci analysis Data for this study were available from a large-scale genetic association study of human gene expression traits in multiple disease-targeted tissue samples including subcutaneous fat, lymphoblastoid cell lines and whole skin, derived from 856 monozygotic (MZ) and dizygotic (DZ) female twins from the TwinsUK cohort, as part of the MuTHER project [18] . We interrogated only lead SNPs (or proxies in LD, r 2 >0.8) using Genevar software [17] . For whole-blood eQTL studies, samples were obtained from a large population-based study [38] . The whole-blood eQTL results were downloaded from the GTex Browser at the Broad Institute on 26 November 2013 [39] . We identified alias rsIDs for significant index SNPs using JLIN software and UK10K WGS data. Associations at P <1 × 10 −3 were considered significant. DNA methylation analysis DNA methylation profiles were obtained in whole-blood samples from 279 MZ and DZ twins from the TwinsUK cohort using the Illumina Infinium HumanMethylation450 BeadChip. Illumina beta values were quantile normalized to a standard normal distribution and corrected for chip, order of the sample on the chip, bisulfite-converted DNA concentration and age. The resulting values were used for meQTL analysis, which was performed separately in two samples, first in 149 unrelated individuals from the TwinsUK WGS sample and second in 130 individuals with deeply imputed data from the TwinsUK GWAS sample. MeQTL analysis was performed for each sample in PLINK by fitting an additive model and meta-analysis across the two samples was performed in GWAMA, where we considered results without strong evidence for heterogeneity (Cochran’s Q P >0.05 and I 2 <0.7). We analysed genotype data at 17 sequence variants (from Table 1 ), where for each variant meQTL analysis was performed with all DNA methylation array CpG sites located within 50 kb of the variant, resulting in 265 pair-wise tests. MeQTL results ( Supplementary Table 8 ) are presented for variants with nominally significant associations in both the WGS and GWAS samples less than a meta-analysis P -value of 1 × 10 −04 . In the PDE8B gene, we also considered meQTL effects at the eQTL rs251429 ( Supplementary Table 7 ) and found nominally significant association with DNA methylation at CpG site cg16461538 ( B =−0.18, s.e.=0.08, P =0.02). We assessed the association between DNA methylation levels at the CpG sites identified to harbour meQTLs in our study ( Supplementary Table 8 ) and TSH and FT4 levels. Using the same study design as that adopted in the meQTL analysis, we obtained no nominally significant association between DNA methylation at the 11 CpG sites ( Supplementary Table 8 ) for TSH or FT4 levels. Subsequent replication of meQTL associations observed in TwinsUK was performed in the ALSPAC cohort for which DNA methylation profiles from whole blood were available in 745 individuals. Here, data were rank transformed to follow the normal distribution and then regressed against batch number. Analyses were also performed using PLINK, adjusting for age, sex, top 10 PCs (genetic) and houseman-estimated cell counts (to account for cellular heterogeneity). Rare variant analysis We conducted GWAS candidate gene (AADAT, ABO, B4GALT6, CAPNS2, CAPZB, DIO1, DIRC3, ELK3, FBXO15, FGF7, FOXA2, FOXE1, GLIS3, HACE1, IGFBP2, IGFBP5, INSR, ITPK1, LHX3, LOC440389/LOC102467146, LPCAT2, MAF, MBIP, MIR1179, NETO1, NFIA, NKX2-3, NR3C2, NRG1, PDE10A, PDE8B, PRDM11, RAPGEF5, SASH1, SIVA1, SLC25A52, SOX9, SYN2 TMEM196, TPO, TTR, VAV3, VEGFA)-based analyses to test for association of the combined effects of rare variants on TSH and FT4 using SKAT-O software [40] . This approach maximizes statistical power by applying both burden-based and SKATs. We used the TwinsUK and ALSPAC WGS data to examine loci with a known association with TSH and FT4. We examined all SNPs within the candidate gene regions, including variants within 50 kb on either side of the gene with MAF <1% down to a MAF of 0.04% (in a cohort), or 0.02% (overall). These analyses used sequential non-overlapping windows each containing 50 SNPs. Association at P <1.55 × 10 −5 (Bonferroni corrected) was considered significant. For the meta-analysis of rare variant data from the WGS cohorts, we used SkatMeta [41] . Polygenic score analysis We conducted polygenic score analyses to test for substantive polygenic effects on TSH and FT4 and for a shared polygenic basis between thyroid traits and a range of related phenotypes including key cardiovascular traits, metabolic, anthropometric, endocrine and bone traits. Polygenic scores have been used to summarize genetic effects for an ensemble of markers that may not individually achieve significance but are relevant to regulation of the trait. The composite score represents an overall genetic signal and can then be used to obtain evidence of a common genetic basis for related disorders [42] . We ranked SNPs by their marginal association with TSH and FT4 using the meta-analysis data set, with TwinsUK samples excluded (leaving N =13,874 for TSH and N =12,561 for FT4). SNPs were thinned to a set of 2,203,581 approximately independent SNPs using the –indep-pairwise option in PLINK with an LD threshold of r 2 >0.2, window size of 5,000 SNPs and step of 1,000 SNPs. On the basis of their associations in the meta-analysis data, SNPs were selected for constructing polygenic scores according to a range of P value thresholds. Scores were then constructed for subjects in the TwinsUK data sets by forming the weighted sum of trait-increasing alleles, with the weights taken as the effect size in the meta-analysis data. To construct polygenic scores, we used 67 SNPs (rs10028213, rs10030849, rs10032216, rs10420008, rs10499559, rs10519227, rs10799824, rs10917469, rs10917477, rs11103377, rs113107469, rs11624776, rs116552240, rs116909374, rs11694732, rs11726248, rs11755845, rs12410532, rs13015993, rs1537424, rs1571583, rs17020124, rs17723470, rs17776563, rs2046045, rs2235544, rs2396084, rs2439302, rs28435578, rs2928167, rs3008034, rs3008043, rs310763, rs334699, rs334725, rs34269820, rs3813582, rs4704397, rs4804416, rs56738967, rs6082762, rs61938844, rs6499766, rs6885099, rs6923866, rs6977660, rs7128207, rs7190187, rs7240777, rs729761, rs73362602, rs73398284, rs737308, rs753760, rs7568039, rs7694879, rs7825175, rs7860634, rs7864322, rs7913135, rs9322817, rs944289, rs9472138, rs9497965, rs965513, rs966423 and rs9915657) that have been shown to be associated with thyroid hormone levels [8] , [10] , [26] . The polygenic score was then tested for association with relevant thyroid and other phenotypes in the TwinsUK sample. Chemogenomic analysis To identify putative thyroxine-responsive genes among the candidate loci ( AADAT , ABO , B4GALT6 , CAPZB , DIO1 , FOXE1 , IGFBP2 , LHX3 , MAF , MBIP , MFAP3L , NR3C2 , NRG1 , PDE10A , PDE8B , QSOX2 , SLC25A52 , SYN2 , TTR and VEGFA ), gene expression data measured in response to levothyroxine treatment in a range of cell lines were retrieved from the Connectivity Map resource [27] . We considered a genome-wide differential expression rank in the top 5th percentile among 22,283 probes as evidence of differential expression. How to cite this article : Taylor, P. N. et al . Whole-genome sequence-based analysis of thyroid function. Nat. Commun. 6:5681 doi: 10.1038/ncomms6681 (2015).